Modelling the influence of photospheric turbulence on solar flare statistics Solar flares stem from the reconnection of twisted magnetic field lines in the solar photosphere. The energy and waiting time distributions of these events follow complex patterns that have been carefully considered in the past and that bear some resemblance with earthquakes and stockmarkets. Here we explore in detail the tangling motion of interacting flux tubes anchored in the plasma and the energy ejections resulting when they recombine. The mechanism for energy accumulation and release in the flow is reminiscent of self-organized criticality. From this model, we suggest the origin for two important and widely studied properties of solar flare statistics, including the time–energy correlations. We first propose that the scale-free energy distribution of solar flares is largely due to the twist exerted by the vorticity of the turbulent photosphere. Second, the long-range temporal and time–energy correlations appear to arise from the tube–tube interactions. The agreement with satellite measurements is encouraging. Parker conjectured that solar flares are driven by the random continuous motion of the footprints of the magnetic field in the photospheric convection [2] , [3] . This conjecture and the experimental observations of power laws in the energy [4] , [5] , [6] , [7] and waiting time [8] , [9] , [10] distributions stimulated a new way of looking at violent bursts. In particular, the fact that the energy distribution is a power law, a property that flares share with diverse physical phenomena [11] , such as avalanches and earthquakes [12] , led to the formulation of flare occurrence models inspired in self-organized criticality (SOC) [13] , [14] , [15] , [16] , [17] , [18] , [19] , [20] , [21] , [22] , [23] . Although these models reproduce the power-law behaviour in the distribution of flare energies, they predict a Poissonian distribution waiting times, which implies that flares result from an uncorrelated process, contrary to experimental observations [8] , [9] , [10] . This point was stressed by Boffetta et al. [8] who, by implementing shell models for turbulence, reproduced the observational power-law decay of the waiting time distribution. However, their exponents are not universal, depending instead on the model parameters. On the basis of a different approach, the waiting time distribution can also be reproduced in terms of a piecewise Poissonian process [24] . More recently, the existence of correlations between flare energies and waiting times has also been investigated [10] , [25] , [26] , [27] . In particular, Lippiello et al. [27] found that the observed time–energy correlations are not simply attributable to obscuration effects. Here, the term obscuration indicates an observational limitation that can be at the origin of the incompleteness of the catalogue, for example, the occurrence of a large flare can hide the detection of smaller flares occurring nearby. An approach more closely inspired in magnetic reconnection was adopted by Hughes et al. [16] , who proposed a dynamical model of solar flares as cascades of reconnecting magnetic loops, with multiple loops that are randomly driven at their footprints and interact with each other. Despite some discrepancy with experimental observations, they showed a relation of the distribution of magnetic loops with a scale-free network, which conceptually supports SOC. The formulation of a theoretical model able to reproduce both the flare statistics and the behaviour of time–energy correlations remains unsolved. A complete model would require a fully developed realistic convection zone, a stratified atmosphere above it and the study of the interplay between magnetic fields and flows. In addition, the model must be three-dimensional, including explicit resistivity to control the reconnection between the colliding magnetic fields. At present, a numerical study of such a model is far out of reach due to the excessive requirement in computing time. On the other end, simplified models considering magnetic reconnections based on a purely statistical approach and neglecting completely the photospheric flow, fail in reproducing a variety of observational data [13] , [14] , [15] , [16] , [17] , [18] , [19] , [20] , [21] , [22] , [23] . In this study, we present an approach that represents a compromise between these two different scenarios. Here, we introduce and study numerically a theoretical model of solar flare occurrence in terms of reconnection of magnetic flux tubes twisted by the photospheric turbulent flow, which reproduces satisfactorily the flare statistics and the behaviour of time–energy correlations. The motion of the tubes in the solar corona is mainly rooted in the photosphere, which is about ~500 km thick, corresponding to an extremely thin layer as compared with the solar radius. Therefore, in the model proposed here, we consider the photospheric flow as a two-dimensional turbulent system following Kolmogorov scaling. Model description The turbulent fluid dynamics of the photosphere is simulated through a lattice Boltzmann model [28] on a square lattice of size L , with a forcing term that specifically reproduces the Kolmogorov energy spectrum regime (see Methods). Anchored in the photospheric flow, the footprints of the magnetic flux tubes follow the local velocity field, and are twisted by the vorticity. The magnetic lines are modelled as lines (see green and pink lines in Fig. 1 ) wrapped around the semi-circular flux tubes (see semi-transparent grey tori in Fig. 1 ), forming, when twisted, a spring-shaped bundle. This representation, which is conceptually consistent with previous realistic models for the kink instability [29] , leads to an explicit relation between the length of the spring and the magnetic energy stored in the corresponding flux tube (see equation (6) in Methods). 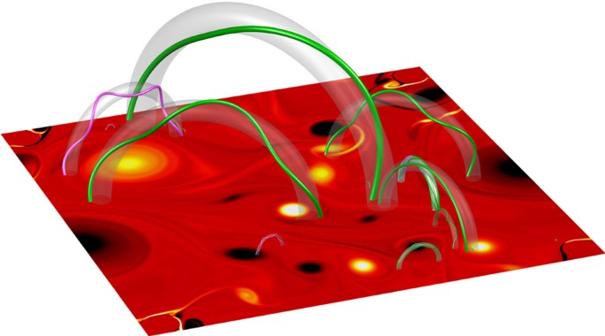Figure 1: Configuration of magnetic tubes in the solar corona. The photospheric plasma is in a turbulent state, where yellow (black) areas denote high (low) vorticity regions. The green and pink lines represent the magnetic lines enclosed in the magnetic flux tubes (semi-transparent grey tori). The pink magnetic lines indicate a magnetic flux tube that has reached the critical twist and, therefore, is at the onset of reconnection, about to release its energy as a flare. Figure 1: Configuration of magnetic tubes in the solar corona. The photospheric plasma is in a turbulent state, where yellow (black) areas denote high (low) vorticity regions. The green and pink lines represent the magnetic lines enclosed in the magnetic flux tubes (semi-transparent grey tori). The pink magnetic lines indicate a magnetic flux tube that has reached the critical twist and, therefore, is at the onset of reconnection, about to release its energy as a flare. Full size image Observational evidence supports the kink instability as the triggering mechanism for magnetic reconnection, and consequently, for solar flare occurrence [30] , [31] , [32] , [33] . The kink instability is an ideal magnetohydrodynamical instability, where magnetic reconnection is not a necessary ingredient, as a flux tube can destabilize by converting twist into writhe. However, in an active region (which is our region of interest), the kink instability will trigger a flare (due to the accumulated free energy), and therefore, we assume that each time a kink instability occurs in a magnetic tube, a flare is released. Accordingly, the kink instability of a flux tube occurs as soon as the intensity of its cumulative twist reaches a given critical value. In our model, the tube releases its total energy (vanishing from the simulation), and a new magnetic flux tube is inserted with the initial condition and located at a random position inside the simulated zone (see Methods). The critical twist Φ c , at which the magnetic reconnection occurs, can be obtained from stability analysis. Several values have been proposed from numerical simulations, theoretical models [29] or deduced from experimental observations [31] , [32] , ranging from 2 π to 12 π , depending on the particular plasma conditions in the corona. Every time a magnetic flux tube reconnects and releases its energy, we implement two possible scenarios: the reconnection heats up the surrounded plasma increasing the local coronal pressure, and therefore, increasing the critical twist of the surrounding magnetic flux tubes [29] . This causes a delay in the reconnection process, which is taken into account here by multiplying the cumulative twist of neighbouring tubes by a positive factor λ R <1, while keeping the critical twist constant. This procedure implements tube–tube interactions and in our simulations we consider either random values or a constant value for λ R , obtaining the same results. Conversely, we also consider the case λ R >1 that induces an avalanching process in the occurrence of solar flares. In this case, every time a magnetic flux tube releases, its energy it increases the twist of the surrounded tubes, triggering new flares and generating a cascade of events. In both cases, the parameter λ R has the important role of tuning the level of tube interactions, whereas non-interacting tubes correspond to λ R =1. We are therefore able to detect how interactions affect the flare waiting time distribution. In what follows, we show that tube–tube interaction is the most relevant ingredient to reproduce the correct temporal organization and the experimentally observed time–energy correlations. We will also show that changing the value of the critical twist within the range of the experimentally meaningful values, does not affect the statistics of solar flares. Our model takes into account the well-known SOC mechanism of slow energy storage by changing the flaring threshold of tubes that are neighbours to the reconnected tube. This mechanism is equivalent to tuning the critical tube twist, a procedure usually implemented in SOC models [13] , [14] , [15] , [16] , [17] , [18] , [19] , [20] , [21] , [22] , [23] . More precisely, by increasing the critical twist ( λ R <1), the photospheric flow has more time to add energy to the respective magnetic flux tubes before they release their energy as a flare. For the case λ R >1, the similarity with SOC models is more evident, since our model can generate a cascade of events by increasing the twist of surrounded magnetic flux tubes, each time a flare is released. Finally, we should mention that our approach does not account for a number of additional features of flare occurrence and flaring active regions [34] , [35] , for example, systematic peculiar flows on top of the heavily suppressed quiet-Sun Kolmogorov flow velocity field, the presence of intense magnetic polarity inversion lines in the photosphere, and slip-running magnetic reconnection in flares. However, the excellent agreement between numerical and observational data suggests that these features are not relevant to produce the observed statistical properties, even if they may be necessary for the complete understanding of solar flares. Peak and total energy distributions Following the described dynamics, the occurrence time and energy released by each flare quantify the statistical properties of our model and are compared with observational data. We perform extensive numerical simulations for different system sizes L =128, 256, 512, 1,024 and 2,048. For each value of L , we first let the fluid evolve without the magnetic flux tubes until it reaches the turbulent regime at Reynolds numbers between 10 4 and 10 5 . The Reynolds number is computed by the relation Re = u rms L / ν , where u rms is the root mean square velocity and ν the kinematic viscosity (values of the Reynolds number and kinematic viscosity for each simulation can be found in the Supplementary Table 1 ). The fully developed turbulence condition is established when the energy spectrum of the flow follows the classical power-law behaviour with Kolmogorov exponent −5/3 (see Supplementary Fig. 1 ). At this point, we add N magnetic flux tubes at random positions and with random initial energies, and record the occurrence time and energy of flares. From previous studies of satellite data by the Solar and Heliospheric Observatory, deviations from the Kolmogorov exponent have been observed depending on the activity of a solar region [36] . However, we show that the choice of the exponent of the spectrum of the turbulent flow does not change appreciably our results (see Supplementary Fig. 2 ). As shown in Fig. 2 , the distribution of peak flare energies follows a typical power-law behaviour, n ( E ) ∝ E − α , with an exponent α =1.68±0.02. As expected, this scaling regime extends up to a cutoff energy that gradually increases with system size L . We compare our results with soft and hard X-ray data from the GOES [37] and the BATSE [38] catalogues, respectively. From the GOES catalogue, only flare events of class C and above (peak flux E > E 0 =10 −6 W m −2 ) observed between 1992 and 2013 are considered, which leads to a total of 19,703 events, covering nearly two solar cycles. In the case of the BATSE catalogue, 7,242 events in the period between 1991 and 2000 were considered, with a peak flux larger than E 0 =0.5 counts s −1 cm −2 . The Kolmogorov–Smirnov test ensures that both samples, numerical and observational data, follow the same scaling behaviour with a P value of 95% (confidence level of 99%). The excellent agreement between numerical and observational data shown in Fig. 2 confirms the validity of the theoretical approach. The exponent of the power law for our numerical results is also in excellent agreement with previous experimental studies [12] , [25] . Notice that in our model for λ R <1, flares are instantaneous events; therefore, we cannot measure separately the peak energy and the total energy associated to each event, or else the energy of a flare is a peak flux energy. Different is the case λ R >1, where avalanching is induced and events are therefore not instantaneous. To implement a unified procedure for models with different λ R , numerical data are compared to peak flux energies from experimental observations. For the case of λ R >1, one can also study the total energy distribution and the duration of each event. In Fig. 3 , we can see that the numerical results are in very good agreement with observations, showing the correct duration and total energy distributions. The exponents for the total energy distribution and the duration of flares, −1.95±0.04 and −3.0±0.1, respectively, are also in good agreement with previous studies [17] . 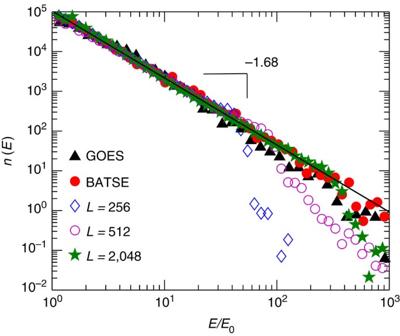Figure 2: Solar flare energies exhibit scale-free behaviour. The distribution of peak flare energies evaluated with our numerical model for different system sizesLandλR<1 shows a power-law regime which increases withL. The solid line is a fit for the largest system size,L=2,048, providing an exponent ofα=1.68±0.02. Observational data from GOES and BATSE catalogues37,38exhibit the same scaling behaviour. Energies are expressed in units of a lower energy cutoff, which isE0=10−6W m−2(GOES) andE0=0.5 counts s−1cm−2(BATSE) for observational data andE0=10 for the numerical catalogues. We have verified that different cutoff values do not affect the scaling behaviour. Figure 2: Solar flare energies exhibit scale-free behaviour. The distribution of peak flare energies evaluated with our numerical model for different system sizes L and λ R <1 shows a power-law regime which increases with L . The solid line is a fit for the largest system size, L =2,048, providing an exponent of α =1.68±0.02. Observational data from GOES and BATSE catalogues [37] , [38] exhibit the same scaling behaviour. Energies are expressed in units of a lower energy cutoff, which is E 0 =10 −6 W m −2 (GOES) and E 0 =0.5 counts s −1 cm −2 (BATSE) for observational data and E 0 =10 for the numerical catalogues. We have verified that different cutoff values do not affect the scaling behaviour. 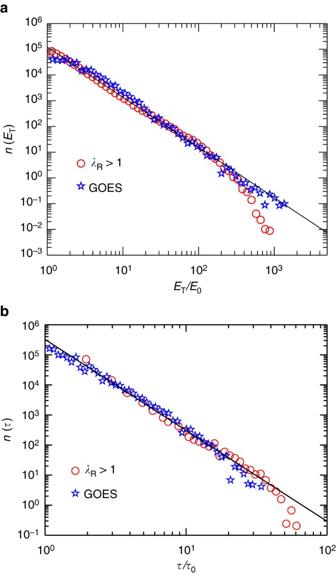Figure 3: Duration of flares and total energy distributions. The distributions of duration of flares and total flare energies are evaluated with our numerical model forλR>1, using a system size ofL=512 andN=400, and compared with observational data from the GOES catalogue37. (a) Total energy distribution. The distribution exhibits a scale-free behaviour with an exponent of −1.95±0.04 (solid line). Energies are expressed in units of a lower energy cutoff, which isE0=6 × 10−7J m−2andE0=11.4 for the observational and numerical data, respectively. (b) Distribution of flare durations. Hereτ0=103s for GOES catalogue andτ0=1 for the numerical data, corresponding to the shortest time at which the power-law regime is observed. The solid line corresponds to an exponent of −3.0±0.1. Full size image Figure 3: Duration of flares and total energy distributions. The distributions of duration of flares and total flare energies are evaluated with our numerical model for λ R >1, using a system size of L =512 and N =400, and compared with observational data from the GOES catalogue [37] . ( a ) Total energy distribution. The distribution exhibits a scale-free behaviour with an exponent of −1.95±0.04 (solid line). Energies are expressed in units of a lower energy cutoff, which is E 0 =6 × 10 −7 J m −2 and E 0 =11.4 for the observational and numerical data, respectively. ( b ) Distribution of flare durations. Here τ 0 =10 3 s for GOES catalogue and τ 0 =1 for the numerical data, corresponding to the shortest time at which the power-law regime is observed. The solid line corresponds to an exponent of −3.0±0.1. Full size image Note that our model results in steeper distribution functions for the total energy than for the peak released energy of the modelled events. On the other hand, numerous observational works report the opposite, that is, clearly flatter distribution functions for the total energy. Theoretical works, at least those relying on SOC, seem also to predict analytically that total energy distributions functions are flatter than those of the peak energy released. Waiting time distributions We also investigate the statistical patterns of the waiting time, defined as the distribution of time delays between the end of an event and the beginning of the next one. As shown in Fig. 4 , the numerical results from our theoretical approach are also in very good agreement with experiments. The distribution is not a simple exponential, suggesting that flare occurrence is not a purely uncorrelated Poisson process. To closely compare the different numerical and observational catalogues, we have rescaled the waiting times, Δ t , by the average event rate in each catalogue [39] , that is, by the inverse of the average waiting time, Λ= N e /( t max − t min ), where N e is the number of events in the respective catalogue. Here t max and t min are the times at which the last and first events in the catalogue occur, respectively. As shown in Fig. 4 , rescaled distributions for numerical and observational data collapse onto a universal curve well fitted by [40] , , where a and b are constants, and α t =2.8±0.2 denotes the exponent of the power-law regime of the distribution for large waiting times. This result is reasonable when compared with previously reported observational values, α t =2.16±0.05 (ref. 39 ) and α t =2.4±0.1 (ref. 7 ). We have also performed the Kolmogorov–Smirnov test, finding that both samples, numerical and observational data, come from the same distribution with a P value of 92% (confidence level of 99%). 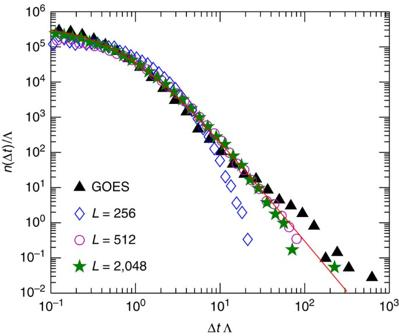Figure 4: Solar flares exhibit a complex temporal organization. The waiting time distribution for solar flares is shown for different system sizesLand compared with observational data for the GOES catalogue37. The distributions indicate that the process is not a simple Poisson process. The solid line denotes the fit for the largest system size,L=2,048, using as a fitting function the analytical expression proposed in ref.39. To better compare the different catalogues, waiting times are normalized by Λ, the average rate evaluated for each numerical and observational catalogue. Figure 4: Solar flares exhibit a complex temporal organization. The waiting time distribution for solar flares is shown for different system sizes L and compared with observational data for the GOES catalogue [37] . The distributions indicate that the process is not a simple Poisson process. The solid line denotes the fit for the largest system size, L =2,048, using as a fitting function the analytical expression proposed in ref. 39 . To better compare the different catalogues, waiting times are normalized by Λ, the average rate evaluated for each numerical and observational catalogue. Full size image It is interesting to investigate the role of different ingredients of the theoretical model on the statistical properties of energy released and waiting times, to identify the main triggering mechanisms for the occurrence of solar flares. We start by considering that, instead of being driven by the turbulent flow, the magnetic flux tubes might move along purely random trajectories and the cumulative twist is calculated by assigning a random vorticity at each footprint. Results in Fig. 5 show that the suppression of the turbulent flow leads to an energy distribution that is exponential rather than a power law. Next, we consider the case where there is a single magnetic flux tube evolving in the turbulent flow, eliminating the possible role of interactions among tubes. We observe in Fig. 5 that the power-law regime in the peak energy distribution is recovered. These two results strongly suggest that the ingredient responsible for the power-law in the energy distribution is the turbulent motion of the footprints anchored into the photosphere, and not tube–tube interactions. We finally consider the case of several tubes having different degree of interaction, that is, either interacting ( λ R <1 and λ R >1) or non-interacting ( λ R =1) tubes. Results shown in Fig. 5 confirm that interactions do not modify the distribution of solar flare energies. Interestingly, models with and without avalanching exhibit the same scaling exponent for the peak flare energy distribution, suggesting that indeed small flares share similar statistical properties with major flares. 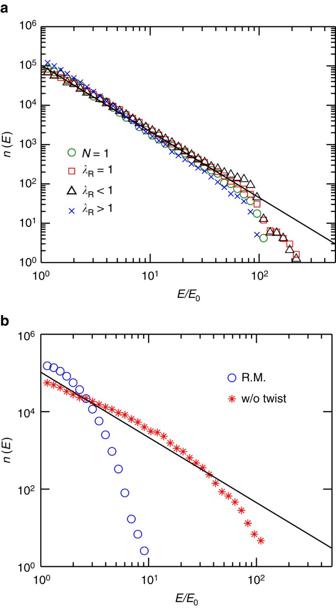Figure 5: Physical ingredients leading to scale-free behaviour for flare energies. Different models are compared to extract the crucial ingredients of the power-law behaviour measured for the energy distribution. The system size isL=512 for all curves. (a) Flare peak energy distribution for simulations where a single flux tube (N=1) evolves in the turbulent flow and reconnects at twisting threshold. The power-law behaviour is recovered with exponentα=1.68±0.02 (solid line). The same behaviour is recovered when changing interactions: from interacting tubes (λR<1 and λR>1) to non-interacting (λR=1) tubes. (b) Solar flare peak energy distribution for the evolution ofN=400 interacting tubes (λR<1) in the case tube footprints diffuse by random motion (denoted by ‘R.M.’). The distribution in this case does not show a power-law regime. For the same system size, we let the tubes evolve according to the turbulent flow but reconnection occurs only through the interaction of footprints or tube crossing (denoted by ‘w/o twist’), that is, twisting of magnetic tubes is not considered. Also in this case, a deviation from the power-law behaviour is observed. The deviations from the power-law regime in both cases are not due to finite-size effects, as can be seen from a systematic finite-size study. The solid line represents the power law obtained for observational data. Results indicate that the turbulent flow and a reconnection ruled by twisting are the ingredients that control energy statistics. Figure 5: Physical ingredients leading to scale-free behaviour for flare energies. Different models are compared to extract the crucial ingredients of the power-law behaviour measured for the energy distribution. The system size is L =512 for all curves. ( a ) Flare peak energy distribution for simulations where a single flux tube ( N =1) evolves in the turbulent flow and reconnects at twisting threshold. The power-law behaviour is recovered with exponent α =1.68±0.02 (solid line). The same behaviour is recovered when changing interactions: from interacting tubes ( λ R <1 and λ R >1) to non-interacting ( λ R =1) tubes. ( b ) Solar flare peak energy distribution for the evolution of N =400 interacting tubes ( λ R <1) in the case tube footprints diffuse by random motion (denoted by ‘R.M.’). The distribution in this case does not show a power-law regime. For the same system size, we let the tubes evolve according to the turbulent flow but reconnection occurs only through the interaction of footprints or tube crossing (denoted by ‘w/o twist’), that is, twisting of magnetic tubes is not considered. Also in this case, a deviation from the power-law behaviour is observed. The deviations from the power-law regime in both cases are not due to finite-size effects, as can be seen from a systematic finite-size study. The solid line represents the power law obtained for observational data. Results indicate that the turbulent flow and a reconnection ruled by twisting are the ingredients that control energy statistics. Full size image We now consider the waiting time distribution for the previous cases. Indeed, in Fig. 6 , we see that the case of random footprint motion and the case of a solitary tube are well described by a Poissonian distribution (dashed line). This implies that, although essential to the recovery of a scale-free energy distribution, the turbulent fluid flow alone is not able to provide the right temporal organization of solar flare occurrence. If more tubes are considered, the distribution starts to deviate from a Poissonian one. For coexisting but non-interacting tubes ( N >1, λ R =1), the turbulent flow in the photosphere is able to induce time correlations between them, although not sufficiently to reproduce the observational results. Indeed, the physical correlations are fully recovered only for interacting tubes ( N >1, λ R <1 and λ R >1). From our results, we can conclude that, whereas the turbulent photospheric flow is the main mechanism responsible for the energy distribution, the interaction between magnetic tubes is what introduces the right temporal correlations in the process. 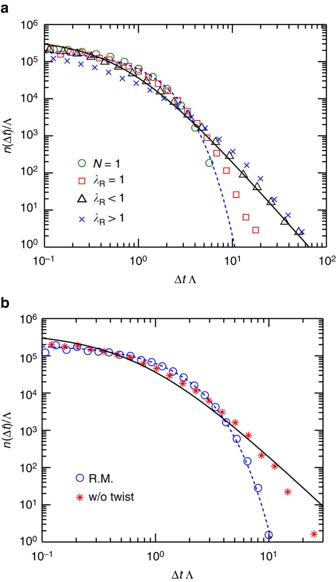Figure 6: Physical ingredients leading to flare organization in time. Different cases are compared to extract the crucial ingredients of the observed waiting time distribution. The system size isL=512 for all curves. (a) Waiting time distribution for simulations where a single flux tube (N=1) evolves in the turbulent flow and reconnects at the twisting threshold. The distribution exhibits an exponential decay (dashed blue line). Conversely, for different degrees of interaction (interacting tubes,λR<1 andλR>1) and non-interacting tubes (λR=1), one recovers the behaviour measured inFig. 4. (b) Distributions evaluated for the evolution ofN=400 tubes in the two cases: Interacting tubes (λR<1), whose footprints diffuse by random motion (denoted by ‘R.M.’) and evolution in the turbulent flow w/o twist. In both cases, deviations from the observational result are observed (the dash blue line denotes an exponential decay). The solid line inaandbrepresents the best fit for the largest system size,L=2,048. Results indicate that tube interactions rule the temporal organization of flares. Figure 6: Physical ingredients leading to flare organization in time. Different cases are compared to extract the crucial ingredients of the observed waiting time distribution. The system size is L =512 for all curves. ( a ) Waiting time distribution for simulations where a single flux tube ( N =1) evolves in the turbulent flow and reconnects at the twisting threshold. The distribution exhibits an exponential decay (dashed blue line). Conversely, for different degrees of interaction (interacting tubes, λ R <1 and λ R >1) and non-interacting tubes ( λ R =1), one recovers the behaviour measured in Fig. 4 . ( b ) Distributions evaluated for the evolution of N =400 tubes in the two cases: Interacting tubes ( λ R <1), whose footprints diffuse by random motion (denoted by ‘R.M.’) and evolution in the turbulent flow w/o twist. In both cases, deviations from the observational result are observed (the dash blue line denotes an exponential decay). The solid line in a and b represents the best fit for the largest system size, L =2,048. Results indicate that tube interactions rule the temporal organization of flares. Full size image Time–energy correlations We further investigate the statistical features of time–energy correlations [27] . For each catalogue, we analyse how the flare energies are organized in time, by evaluating the probability that a flare with energy E i is followed by a flare with energy larger than λE i under the conditions that their temporal distance Δ t is smaller than a certain threshold t th , P ( λ | t th )= P ( E i +1 / E i > λ |Δ t i < t th ). For each catalogue, this probability fluctuates wildly due to statistical noise. Therefore, to eliminate this noise, we evaluate the same probability also in a synthetic catalogue generated by reshuffling the flare energies with respect to their occurrence time, such that energy and time are uncorrelated by construction. We then consider the difference between the conditional probabilities, δP ( λ | t th ), evaluated in the two data sets. This difference is different from zero only if significant time–energy correlations are present in the original catalogue. In particular, if | δP ( λ | t th )| is larger than zero, it is more likely to find two consecutive flares satisfying both conditions ( E i +1 / E i > λ and Δ t i < t th ) in the real rather than in the reshuffled catalogue (see Methods). By using the same technique, we also compute the conditional probability difference δP ( E th | t th ) to observe a flare energy larger than a given threshold E th after an waiting time smaller than t th . We consider the behaviour of both conditional probability differences for a range of parameters λ , t th and E th . In Fig. 7 , we see that the probability differences are very well described by our model with λ R <1. In particular, for both, numerical and observational results, δP ( λ | t th ) is different from zero beyond error bars. This implies that it is very likely that for close-in-time flares the second one will have slightly larger energy than the previous one (the maximum is for ), as far as their separation in time is shorter than approximately 25 h. These energy correlations decrease as the temporal separation increases. Conversely, it is very unlikely to observe in real catalogues close-in-time flares where the second one has a smaller energy ( δP <0 for ( λ <1)). Furthermore, in Fig. 7b , curves for δP ( E th | t th ) are different from zero beyond error bars and decrease with increasing t th . This implies that the probability to find couples of successive flares with the second flare having energy higher than E th decreases, if one includes events separated by a larger Δ t in the analysis. For large E th , numerical results deviate from the observational ones. This can be due to the finite size of our simulation, which imposes an upper limit to the flux tube sizes, and therefore limits the maximum energy of flares (see also Fig. 2 , where finite-size effects in the energy distribution are analysed). Note that the agreement between observational and numerical data is very good, suggesting that, in fact, the turbulent flow and magnetic flux tube interactions induce correlations between energy and time in the occurrence of solar flares. 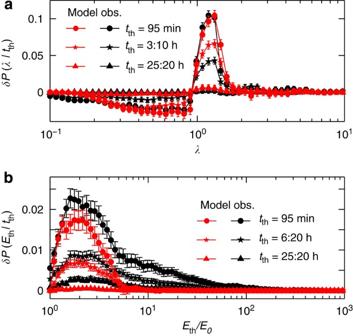Figure 7: Flare energies and occurrence times are correlated. (a) The conditional probability differenceδP(λ|tth)=δP(Ei+1/Ei>λ|Δti<tth) is plotted as function of the parameterλfor differenttth. Black and red colours represent the observational and numerical catalogues, respectively. Error bars report the s.d. of the probability evaluated for the reshuffled catalogue (see Methods).δPis different from zero beyond error bars for a range ofλ>1 indicating that, both in the observational and numerical catalogue, for consecutive flares occurring within 3 h the energy of the second flare is larger than the energy of the previous flare. (b) The conditional probability differenceδP(Eth|tth)=δP(Ei+1>Eth|Δti<tth) as function of the energy thresholdEthfor differenttth. To compare the different catalogues, energies are normalized byE0=1.5 × 10−6W m−2for observational data andE0=150 for numerical data.δPis different from zero beyond error bars for energy thresholdsEthup to about 10E0indicating that, both in the observational and numerical catalogue, as consecutive flares become more distant in time, the probability to find the following flare with energy higher thanEthbecomes smaller. To convert the numerical units of time, Δtnum, into physical units, Δt, we have used the expression Δtnum=ΛΔt/Λn, where Λnand Λ are the inverse of the average waiting times for the numerical and observational catalogues, respectively. Figure 7: Flare energies and occurrence times are correlated. ( a ) The conditional probability difference δP ( λ | t th )= δP ( E i +1 / E i > λ |Δ t i < t th ) is plotted as function of the parameter λ for different t th . Black and red colours represent the observational and numerical catalogues, respectively. Error bars report the s.d. of the probability evaluated for the reshuffled catalogue (see Methods). δP is different from zero beyond error bars for a range of λ >1 indicating that, both in the observational and numerical catalogue, for consecutive flares occurring within 3 h the energy of the second flare is larger than the energy of the previous flare. ( b ) The conditional probability difference δP ( E th | t th )= δP ( E i +1 > E th |Δ t i < t th ) as function of the energy threshold E th for different t th . To compare the different catalogues, energies are normalized by E 0 =1.5 × 10 −6 W m −2 for observational data and E 0 =150 for numerical data. δP is different from zero beyond error bars for energy thresholds E th up to about 10 E 0 indicating that, both in the observational and numerical catalogue, as consecutive flares become more distant in time, the probability to find the following flare with energy higher than E th becomes smaller. To convert the numerical units of time, Δ t num , into physical units, Δ t , we have used the expression Δ t num =ΛΔ t /Λ n , where Λ n and Λ are the inverse of the average waiting times for the numerical and observational catalogues, respectively. Full size image It is important to notice that agreement with observational data is only obtained for interacting tubes ( λ R <1), not for non-interacting tubes, single tube and random motion of tube footprints, where δP ( E th | t th ) ≃ 0 and δP (λ| t th ) ≃ 0 are found. For the case λ R >1, we do not obtain full quantitative agreement with time–energy correlations measured in experimental catalogues (see Fig. 8 ). Data still predict that the next flare statistically has slightly larger energy than the previous one but in a narrower λ range and with a smaller probability. Moreover, the case λ R >1 is not able to reproduce the anticorrelations for λ <1. These results suggest that the relaxation mechanism corresponding to λ R <1 seems to be more appropriate to reproduce time–energy interaction, as compared with the avalanche process characterized by λ R >1. 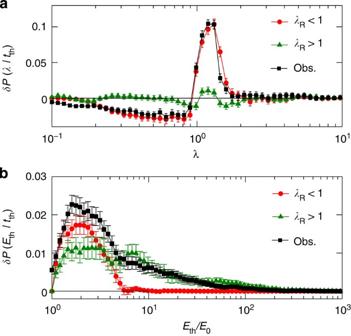Figure 8: Physical ingredients leading to time–energy correlations. (a) The conditional probability differenceδP(λ|tth) is plotted as function of the parameterλfortth=95 min. Error bars report the s.d. of the probability evaluated for the reshuffled catalogue (see Methods). For the caseλR<1,δPis different from zero beyond error bars and in quantitative agreement with observational data. Conversely, for the case λR>1,δP>0 in a narrow range, with an amplitude in disagreement with correlations measured in catalogues. (b) The conditional probability differenceδP(Eth|tth) as function of the energy thresholdEthfor both interacting models,λR>1 andλR<1. To compare the different catalogues, energies are normalized byE0=150 for both catalogues.δPis different from zero beyond error bars for energy thresholdsEthup to about 10E0(forλR<1) and 100E0(forλR>1) indicating that, both models can reproduce this kind of correlations. For computing the conditional probabilities, we have chosentth=95 min. By increasingtth, we recover, for both catalogues, that the time–energy correlations decrease as inFig. 7. Figure 8: Physical ingredients leading to time–energy correlations. ( a ) The conditional probability difference δP ( λ | t th ) is plotted as function of the parameter λ for t th =95 min. Error bars report the s.d. of the probability evaluated for the reshuffled catalogue (see Methods). For the case λ R <1, δP is different from zero beyond error bars and in quantitative agreement with observational data. Conversely, for the case λ R >1, δP >0 in a narrow range, with an amplitude in disagreement with correlations measured in catalogues. ( b ) The conditional probability difference δP ( E th | t th ) as function of the energy threshold E th for both interacting models, λ R >1 and λ R <1. To compare the different catalogues, energies are normalized by E 0 =150 for both catalogues. δP is different from zero beyond error bars for energy thresholds E th up to about 10 E 0 (for λ R <1) and 100 E 0 (for λ R >1) indicating that, both models can reproduce this kind of correlations. For computing the conditional probabilities, we have chosen t th =95 min. By increasing t th , we recover, for both catalogues, that the time–energy correlations decrease as in Fig. 7 . Full size image Finally, we have performed extensive simulations varying every parameter of the model, namely, the critical twist Φ c , the magnetic flux tube density via N and the size ratio of the magnetic flux tubes r c / R (where r c and R are the inner and outer radii of the magnetic flux tubes). For all cases, results for flare statistics and time–energy correlations remain unchanged as shown in the Supplementary Figs 3–5 . It is well accepted in the literature that solar flare occurrence is a process driven by magnetic reconnection. Since high-quality satellite data became accessible, several studies have evidenced that the statistics of this phenomenon is complex: it exhibits scale-free energy distribution and a nontrivial waiting time distribution. A number of theoretical models attempted to reproduce such statistics with different approaches. This study implements magnetic reconnection in a model framework that enables us to test the role of the different physical ingredients on observed statistical patterns. In particular, we have shown that the energy distribution are ruled by the turbulent features of the flow in the photospheric plasma. More precisely, that, if tube footprints simply diffuse in the corona in absence of turbulent flow, the observed distribution of flare energies would be exponential, namely it would exhibit a characteristic flare size. Moreover, the turbulent flow alone is not sufficient to fully reproduce the statistical patterns of real data. Indeed the evolution of a single tube or several non-interacting tubes in the corona, exhibiting the observed energy distribution, is not sufficient to account for temporal correlations. The detailed analysis of the energy organization in time indicates that turbulence and tube interactions are the essential physical ingredients controlling solar flare occurrence. Proving time–energy correlations is the first step towards any forecasting model. This could be formalized by implementing the phenomenological laws, as done for earthquakes [41] (ETAS model), and would open a novel field of investigation. Evaluation of the turbulent flow For modelling the two-dimensional turbulent flow, we have used a two-dimensional lattice Boltzmann model of size L with a cell configuration D 2 Q 9 (2 dimensions and 9 discrete velocity vectors) [28] . To induce turbulence, we have included the following forcing term in the 2D Navier–Stokes equation where A 0 is a constant, k f =2 πq and q varies in time such that each value of q is used during an interval of time s =(4 q / L ) − μ , and then is increased by one. As an initial value, we take q =2. Here, μ is a tuning parameter to control the spectrum of the energy of the turbulent flow (in our simulations, μ =5/3). The coefficient 4 defines the minimum wave number (due to space discretization limitations). This forcing term satisfies the incompressibility condition ∇ F =0. The kinematic viscosity of the fluid is set to ν =10 −3 and the forcing coefficient to A 0 =10 −8 . As initial conditions for the fluid, we choose density ρ =1, and velocity u =(0,0). Furthermore, we also impose a large-scale dissipation mechanism to avoid vortex condensation [42] . All the values are in numerical units. Once the fluid has reached the turbulent regime, we insert N magnetic flux tubes in random positions. The position of the respective footprints for each tube l , denoted by x l + for the positive footprint and x l − for the negative one, is a function of time and evolves as, where u ( x ) is the velocity of the fluid at position x . Then, we can define w l + and w l − as the cumulative twist in the positive and negative footprint, respectively, evolving according to the equation, Note that the component used to twist the magnetic flux tubes is the z-component of the vorticity, since the velocity lies on the two-dimensional space. As initial conditions, the flux tubes have an outer radius of R =4 cells and zero twist, w l ± =0. If the positive footprint of a tube comes very close to its negative partner (less than two lattice nodes), we reset the tube to the initial condition (initial length and zero twist) and relocate it at a random position inside the simulated zone. The vanishing of these tubes can be seen as small reconnection processes with negligible released energy. Because of space discretization in our numerical simulations, the position of each footprint is, in general, not located at a fluid grid point, therefore we use bilinear interpolation to calculate the velocity at the footprint position. Note that the motion of the footprints, see equation (2), as well as the twist, see equation (3), are additive (See Supplementary Fig. 6 ), in the sense that they systematically inject electric currents and associated magnetic energy in the system. The magnetic field lines are modelled as lines wrapped around semi-circular flux tubes, forming, when twisted, a spring-shaped bundle (see Fig. 1 ). Therefore, we can assume that the total energy of a tube is given by the length of the magnetic line, which depends on the twisting and the size of the semi-circular tube. Thus, when a flux tube is not twisted, its energy equals E l = πR (here and throughout the following calculation, we have omitted the proportionality constant to get the right units of energy). On the other hand, if a flux tube is twisted, the spring-shaped bundle can be parametrized by where r c is the cross-section radius of the semi-circular tube. The value ξ depends on ω as follows: ξ =Θ ω , where Θ is a constant that controls the number of turns that the magnetic line makes around the semi-circular tube. In this coordinate system ( x , y , z ), the photosphere is located at the plane x − y . The length of this parametric curve is given by the integral, According to the kink instability theory [29] , the twist is defined as Φ = πRB θ / r c B z , where B θ and B z are the tangential and perpendicular components of the magnetic field to the plane x − y at the footprint ( ω =0). Therefore, the ratio B θ / B z is equivalent to the ratio between the y and z components of the derivative of the parametric curve, B θ / B z =( dR ly / dω )/( dR lz / dω ) with ω =0, and we can conclude that Φ = πR Θ/(2 r c + R ) is the twist. In our model, Θ denotes the cumulative total angle due to the vorticity of the fluid, Θ= w l + + w l − . The integral in equation (5) does not possess an analytical solution. However, we can assume that r c ≪ R , obtaining a very simple expression: Note that this expression is identical to the expression for an untwisted flux tube for any values of r c and R . Once a magnetic flux tube reaches the critical twist Φ c , the tube releases its entire energy and vanishes. To keep the tube density in a stationary state and produce a sufficient statistics, a new tube is placed at a random position inside the simulated zone with the initial condition ( w l ± =0 and R =4 cells). When several magnetic flux tubes reach the critical twist within the same temporal interval δt =1, we sum the energies of the tubes into a single event. For the case λ R <1, we have also evaluated the distributions keeping simultaneous events separate (see Supplementary Fig. 5 ) and verified that the main properties of solar flare statistics remain unchanged. For the case of λ R >1, since flaring occurs through an avalanching process, we perform the measurement of events as follows. Once a flare occurs, we stop the fluid and observe if it triggers other flares. We measure the peak flux energy as the largest flare that occurs within the avalanche process, and the total energy as the sum of all flares. The duration of flares is taken as the total number of released flares. Afterwards, the dynamics of the photospheric flow is restarted. Our model cannot accommodate helicity conservation during the magnetic reconnection process [42] . Therefore, it is assumed that each helical kink instability ejects the unstable flux tube out of the simulation volume to infinity (physically, that would mean that each flare is eruptive). However, it seems that this effect is not relevant to reproduce the solar flare statistics. Note that the energy stored by a tube scales with the tube length and therefore has an upper cutoff controlled by the system size. We have also run the simulations for different initial conditions, finding that our statistical results remain unchanged. In particular, for the cases where r c / R <1 (but not necessarily r c / R ≪ 1), we have solved numerically the integral in equation (5) considering terms up to order ( r c / R ) 10 . We have implemented our numerical code using CUDA C. The simulations for a fixed set of parameters run 3 weeks on a cluster of 12 graphic cards, Nvidia Tesla M2075, each one containing 448 GPU cores. Conditional probability analysis Each flare i in the numerical and observational catalogues is characterized by its starting time t i and its peak flux energy E i . From each catalogue, we evaluate the conditional probability P ( λ | t th )= P ( E i +1 / E i > λ |Δ t i < t th ) to find the energy of the next flare ( E i +1 ) being larger than λ times the energy of the previous flare ( E i ), if their temporal distance, Δ t ≡ t i +1 − t i , is smaller than a certain threshold, t th . For comparison, the same conditional probability is evaluated from a reshuffled sequence of the same energy–time series. In such synthetic catalogues, we expect that flare energies and occurrence times are totally uncorrelated. Keeping λ and t th fixed, we compute the quantity P *( λ | t th ) for 10 5 independent realizations of the reshuffled catalogue, obtaining an ensemble of values which follows a Gaussian distribution with mean value Q ( λ | t th ) and s.d. σ ( λ | t th ). We then define δP ( λ | t th )≡ P ( λ | t th )− Q ( λ | t th ). If the absolute value | δP ( λ | t th )|> σ ( λ | t th ), a significant difference in the number of pairs of sequential energies ( E i , E i +1 ) satisfying both conditions exists between the real and the reshuffled catalogue. By using the same technique, we also compute the conditional probability difference δP ( E th | t th )≡ P ( E i +1 > E th |Δ t i < t th )− Q ( E th , t th ). How to cite this article: Mendoza, M. et al. Modelling the influence of photospheric turbulence on solar flare statistics. Nat. Commun. 5:5035 doi: 10.1038/ncomms6035 (2014).